Opposing calcium-dependent signalling pathways control skeletal muscle differentiation by regulating a chromatin remodelling enzyme Calcium signalling is important for differentiation-dependent gene expression, but is also involved in other cellular functions. Therefore, mechanisms must exist to distinguish calcium signalling relevant to differentiation. Calcineurin is a calcium-regulated phosphatase that is required for myogenic gene expression and skeletal muscle differentiation. Here, we demonstrate that inhibition of calcineurin blocks chromatin remodelling and that the Brg1 ATPase of the SWI/SNF chromatin remodelling enzyme, which is required for the activation of myogenic gene expression, is a calcineurin substrate. Furthermore, we identify the calcium-regulated classical protein kinase C β (PKCβ) as a repressor of myogenesis and as the enzyme that opposes calcineurin function. Replacement of endogenous Brg1 with a phosphomimetic mutant in primary myoblasts inhibits myogenesis, whereas replacement with a non-phosphorylatable mutant allows myogenesis despite inhibition of calcineurin signalling, demonstrating the functionality of calcineurin/PKC-modified residues. Thus, the Brg1 chromatin remodelling enzyme integrates two antagonistic calcium-dependent signalling pathways that control myogenic differentiation. ATP-dependent SWI tch/ S ucrose N on F ermentable (SWI/SNF) chromatin remodelling enzymes are large, multi-protein complexes that are capable of rendering a closed, repressive chromatin structure into an open, transcriptionally competent configuration by altering contacts between DNA and histones [1] . SWI/SNF activity is required for the activation of a large number of genes during development, and has also been implicated in basic cellular functions including replication [2] , [3] and DNA repair [4] . Mutations in SWI/SNF components have been shown to occur frequently in various cancers [5] , [6] , and have also been implicated in other human diseases [7] . Given the broad range of functions for SWI/SNF, the activity of the complex must be regulated in such a way as to direct its activity both spatially and temporally. One mechanism by which this can be accomplished is by changing the properties of SWI/SNF through its specific subunit composition. Variations in subunit composition have been shown to be important for specific developmental programmes, including myogenesis [8] , [9] . However, selection of the catalytic subunit, which can be Brahma (Brm) or Brahma Related Gene 1 (Brg1), provides the most striking difference in function. The two ATPases have similar chromatin remodelling activities in vitro [10] , but mouse modelling approaches have demonstrated that Brg1 is necessary for early embryogenesis and most tissue differentiation events [11] , [12] , [13] , whereas Brm knockout mice exhibited no clear defects [14] . Subunit composition alone, however, cannot fully explain how SWI/SNF enzymes are coordinated to remodel chromatin at specific chromosomal loci in response to signalling cues. To accomplish this, SWI/SNF enzymes likely are responsive to signal transduction through post-translational modification. Indeed, most of the subunits are phosphoproteins [15] , and phosphorylation of the SWI/SNF subunit Baf60c by the p38 mitogen-activated protein kinase is required for the assembly of the enzyme complex at myogenic promoters [8] , [16] . Given the diversity of SWI/SNF subunit composition and the potential for significant post-translational modification, clear evidence for the enzyme complex as a target of multiple signal transduction pathways would identify chromatin remodelling as a key step in translating widely used signal transduction pathways into diverse but specific transcriptional responses. The calcium-sensitive serine/threonine phosphatase calcineurin has been shown to be necessary for differentiation of immortalized rat and primary human myoblasts and for regeneration of damaged muscle in mice in-vivo [17] , [18] . Calcineurin function via control of the sub-cellular localization of the NFAT transcription factor is well-established in other tissue types [19] . However, prior work has revealed a more complicated role for calcineurin in skeletal muscle that likely involves other, yet uncharacterized mechanisms of action [20] . More recent studies showing an interaction of SWI/SNF with calmodulin, a component of calcineurin, and a calcium-dependent step in SWI/SNF-mediated chromatin remodelling [21] raised the possibility that SWI/SNF enzyme might be a target of calcineurin. Because both calcineurin and SWI/SNF have been shown to be required for activation of genes in muscle differentiation, we investigated connections between calcineurin and SWI/SNF enzymes. We show that inhibition of calcineurin blocks chromatin remodelling, myogenic gene expression and myogenic differentiation. We identify protein kinase C βI (PKCβI) as a repressor of myogenesis and as the kinase that opposes calcineurin function. These enzymes temporally regulate the phosphorylation state of the Brg1 ATPase that controls SWI/SNF chromatin remodelling enzyme activity. This work supports the novel conclusion that SWI/SNF enzyme acts as an integrator for two opposing calcium-sensitive pathways, the balance of which regulates skeletal muscle differentiation. Calcineurin regulates Brg1 during myogenic differentiation We sought to investigate whether calcineurin signalling impacted SWI/SNF chromatin remodelling function and its essential role in skeletal myogenesis. First, we verified that inhibition of calcineurin, either with the drug FK506 (ref. 22 ) or by overexpression of the calcineurin inhibitory peptide (CAIN) [23] , blocked differentiation of C2C12 myoblasts and induction of myogenin ( Supplementary Fig. 1a ) and Myosin Heavy Chain (MyHC, Supplementary Fig. 1b ), without altering levels of MyoD ( Supplementary Fig. 1c ). Because it is difficult to separate the effect of loss of myogenin activity and possible effects of calcineurin on the later stages of myogenic gene expression, which are myogenin dependent, we focused our search for additional targets of calcineurin on the myogenin promoter. It is known that Brg1 remodels chromatin to facilitate myogenin activation [24] , [25] and that Brg1 is inactivated by hyper-phosphorylation during mitosis [26] , making it a potential target for activation by phosphatase activity. We therefore examined the Brg1-dependent chromatin remodelling of the myogenin promoter in the presence of FK506, and found that inhibition of calcineurin activity by FK506 led to a loss of chromatin remodelling activity ( Fig. 1a ) as well as loss of Brg1 binding at the myogenin promoter ( Fig. 1b ), suggesting that calcineurin activity is required for the interaction of the SWI/SNF ATPase with chromatin in differentiating cells. Furthermore, reciprocal co-immunoprecipitations (co-IPs) showed an interaction between calcineurin and the Brg1-containing SWI/SNF complex ( Fig. 1c ). 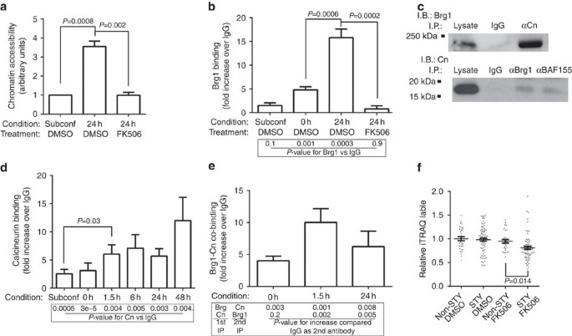Figure 1: BRG1 is a calcineurin target. (a) 24 h post differentiation, the accessibility of a PvuII site in the myogenin promoter increased as measured by restriction enzyme accessibility. In the presence of FK506, this increase in accessibility was lost.P-values were determined by a two-tailed unpairedt-test. (b) ChIP showed that binding of Brg1 to the myogenin promoter occurred after cells became confluent, increased during differentiation and was lost upon FK506 treatment.P-values below the graph indicate the significance of the increase over IgG control using a one-tailed paired ratiot-test;P-values above represent significant differences in the magnitude of binding (Brg1/IgG) as determined by a two-tailed unpairedt-test. (c) Reciprocal co-IPs showed that a calcineurin antibody immunoprecipitated Brg1, and antibodies against SWI/SNF subunits precipitated calcineurin from differentiating C2C12 lysates. (d) ChIP demonstrating that calcineurin bound to the myogenin promoter at all time points tested, as shown by a significant increase in binding compared with IgG (P-values as described inaare shown below the graph). By 1.5 h post differentiation, there was a further increase in calcineurin binding (two-tailed unpairedt-test). (e) Sequential ChIPs (re-ChIPs) showed co-occupancy by Brg1 and calcineurin by 1.5 h post differentiation. The graph shows the results for the Brg1 then Cn re-ChIP.P-values shown beneath the graph are one-tailed paired ratiot-tests for an increase in binding using the antibody orders described compared with control samples immunoprecipitated with IgG as the second antibody. Data in quantified experiments reflect averages of three independent experiments each run in duplicate ±s.d. (f) Using differential iTRAQ labelling, the abundance of each non-modified peptide obtained from trypsin-digested Brg1 isolated from differentiating C2C12 cells was compared with the abundance of the same sequence present in the half of the sample that had been subjected toin vitrodephosphorylation. This indirectly provides quantification of the phosphorylated fraction of each peptide. Brg1 from DMSO-treated cells showed equivalent ratios of isobaric labelling between non-phosphorylatable (non-STY) and phosphorylatable (STY) peptides. Using a two-tailedt-test, Brg1 from FK506-treated cells showed a statistically significant difference between these two groups, indicating hyperphosphorylation of Brg1 in the absence of calcineurin activity. Figure 1: BRG1 is a calcineurin target. ( a ) 24 h post differentiation, the accessibility of a PvuII site in the myogenin promoter increased as measured by restriction enzyme accessibility. In the presence of FK506, this increase in accessibility was lost. P -values were determined by a two-tailed unpaired t -test. ( b ) ChIP showed that binding of Brg1 to the myogenin promoter occurred after cells became confluent, increased during differentiation and was lost upon FK506 treatment. P -values below the graph indicate the significance of the increase over IgG control using a one-tailed paired ratio t -test; P -values above represent significant differences in the magnitude of binding (Brg1/IgG) as determined by a two-tailed unpaired t -test. ( c ) Reciprocal co-IPs showed that a calcineurin antibody immunoprecipitated Brg1, and antibodies against SWI/SNF subunits precipitated calcineurin from differentiating C2C12 lysates. ( d ) ChIP demonstrating that calcineurin bound to the myogenin promoter at all time points tested, as shown by a significant increase in binding compared with IgG ( P -values as described in a are shown below the graph). By 1.5 h post differentiation, there was a further increase in calcineurin binding (two-tailed unpaired t -test). ( e ) Sequential ChIPs (re-ChIPs) showed co-occupancy by Brg1 and calcineurin by 1.5 h post differentiation. The graph shows the results for the Brg1 then Cn re-ChIP. P -values shown beneath the graph are one-tailed paired ratio t -tests for an increase in binding using the antibody orders described compared with control samples immunoprecipitated with IgG as the second antibody. Data in quantified experiments reflect averages of three independent experiments each run in duplicate ±s.d. ( f ) Using differential iTRAQ labelling, the abundance of each non-modified peptide obtained from trypsin-digested Brg1 isolated from differentiating C2C12 cells was compared with the abundance of the same sequence present in the half of the sample that had been subjected to in vitro dephosphorylation. This indirectly provides quantification of the phosphorylated fraction of each peptide. Brg1 from DMSO-treated cells showed equivalent ratios of isobaric labelling between non-phosphorylatable (non-STY) and phosphorylatable (STY) peptides. Using a two-tailed t -test, Brg1 from FK506-treated cells showed a statistically significant difference between these two groups, indicating hyperphosphorylation of Brg1 in the absence of calcineurin activity. Full size image Because Brg1 is a nuclear protein, interaction with calcineurin should occur within the nucleus. Epifluorescent images of confluent C2C12 cells stained for calcineurin showed cytoplasmic staining with nuclear foci ( Supplementary Fig. 2a ). Addition of Leptomycin B resulted in nuclear accumulation, demonstrating active shuttling of calcineurin between the nucleus and the cytoplasm ( Supplementary Fig. 2b ). Some co-localization of Brg1 and calcineurin in nuclear foci was observed ( Supplementary Fig. 2c,d ), supporting the co-IP data. We also investigated Brg1 and calcineurin co-localization in sub-confluent proliferating cells, but saw no clear difference from the co-localization seen in confluent cells ( Supplementary Fig. 2e ). These data raised the possibility that calcineurin is capable of binding chromatin. Chromatin immunoprecipitation (ChIP) experiments showed that calcineurin was bound to the myogenin promoter even in proliferating cells ( Fig. 1d ) as shown by a significant increase in pull-down compared with the IgG control. Calcineurin binding increased soon after differentiation began ( Fig. 1d ; 1.5 h). This increase in binding corresponded to co-occupation of the promoter by both calcineurin and Brg1 as shown by sequential, or re-ChIP, experiments ( Fig. 1e ), suggesting that the two proteins form a stable complex on chromatin in differentiating cells. As calcineurin is a phosphatase, it is expected that a target protein would be hyperphosphorylated in cells treated with a calcineurin inhibitor. To examine calcineurin-sensitive Brg1 phosphorylation, we utilized an indirect mass spectrometry (MS) method that allows for inference of a peptide’s phosphorylation state ( Supplementary Fig. 3a ) [27] . Using this method on immunoprecipitated Brg1, tryptic peptides covering 31.6% of the length of Brg1 were identified ( Supplementary Table 1 ). Analysis of the phosphorylation state of Brg1 revealed that peptides from dimethylsulphoxide (DMSO)-treated cells showed no differences between potentially phosphorylated peptides (those containing serine, threonine or tyrosine (STY)) and those that cannot be phosphorylated (non-STY)). However, peptides from Brg1 isolated from FK506-treated cells showed a significant difference in labelling between STY and non-STY peptides, suggesting hyper-phosphorylation in the absence of calcineurin activity ( Fig. 1f ). PKCβI phosphorylates Brg1 and represses myogenesis The MS data were then used to predict which kinase might be responsible for Brg1 hyperphosphorylation in the FK506-treated sample. For each peptide, the likely presence or absence of a site for 16 different kinases was determined using NetPhosK [28] . The kinase predictions for protein kinase C (PKC) are included in Supplementary Table 1 (right-most column). We then used the relative abundance of the non-phosphorylated peptide divided by the total amount of peptide as an indication of the extent of phosphorylation of each peptide. When the peptides were sorted by phosphorylation score (columns 7 and 9, Supplementary Table 1 ), those with potential PKC sites clustered near the top of the list ( Supplementary Fig. 3b ). We performed a logistic regression to look for an association between peptide phosphorylation and the predicted presence of a kinase site as identified by NetPhosK [28] . There was a statistically significant association for PKC ( P =0.04), but not for any of the other kinases examined ( Supplementary Fig. 3b ). This suggests that PKC might be a kinase involved in Brg1 phosphorylation. We note that had we obtained greater coverage of Brg1, it is likely that additional kinases would have been identified as candidate kinases. This should be expected, as Brg1 has long been known as a heavily phosphorylated protein [26] , [29] , [30] , not all peptides that we detected were sensitive to the calcineurin inhibitor, suggesting that other phosphatases and perhaps other kinases are relevant, and indeed other kinases have been implicated as regulating Brg1 phosphorylation [26] , [29] . If PKC is responsible for phosphorylating calcineurin target sequences, then inhibition of PKC should relieve the repression of myogenesis caused by calcineurin inhibition. We found that the drug Go6976, which inhibits the activity of the calcium-sensitive classical PKC isoforms [31] , restored both myogenin ( Fig. 2a,b ) and MyHC ( Fig. 2c,d ) expression in cells treated with FK506 or in cells overexpressing CAIN ( Supplementary Fig. 4a ). In addition, the expression of other marker genes, including acetylcholine receptor and Caveolin 3, confirmed that FK506 sensitivity was reversed by treatment with Go6976 ( Fig. 2e,f ). These results indicate for the first time that the calcium-sensitive PKCs inhibit myogenesis, and that an additional calcium-dependent signal, calcineurin, is required to relieve this repression. 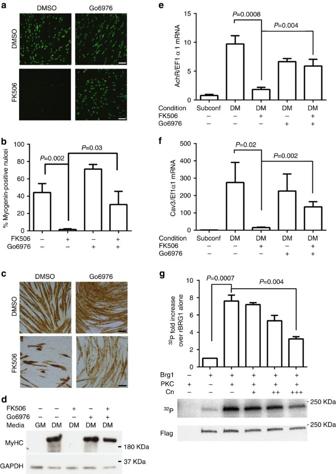Figure 2: PKC antagonizes calcineurin function. (a,b) The classical PKC inhibitor Go6976 restored myogenin expression in FK506-treated C2C12 cells as shown by immunofluorescence staining and confirmed by counting of stained nuclei. Five fields for each sample were counted for each of three independent experiments. Data represent the average ±s.d.P-values were determined by a two-tailedt-test. Size bars, 100 μm. (c,d) Myosin heavy chain (MyHC) expression was similarly restored as shown by immunocytochemistry and western blotting. Size bars, 100 μm. (e,f) Inhibition of classical PKC activity by treatment with Go6976 rescued mRNA expression of additional myogenic genes, including acetylcholine receptor (AchR) and Caveolin 3 (Cav3). The data represent the average of three independent experiments each run in triplicate ±standard deviation. The values from the subconfluent (Subconf) samples were set to 1. TheP-values represent two-tailedt-tests for differences between samples indicated. (g) PKC phosphorylated recombinant FLAG-tagged Brg1 as shown by32P autoradiography. Calcineurin addition inhibited Brg1 phosphorylation by PKC. Quantified data represent the average of three independent experiments ±standard deviation. Two-tailedt-tests showed a significant increase in phosphorylation when Brg1 was treated with PKC, and this phosphorylation decreased when calcineurin was added. A western showing equal loading of FLAG-Brg1 is displayed below the autoradiograph. Figure 2: PKC antagonizes calcineurin function. ( a , b ) The classical PKC inhibitor Go6976 restored myogenin expression in FK506-treated C2C12 cells as shown by immunofluorescence staining and confirmed by counting of stained nuclei. Five fields for each sample were counted for each of three independent experiments. Data represent the average ±s.d. P -values were determined by a two-tailed t -test. Size bars, 100 μm. ( c , d ) Myosin heavy chain (MyHC) expression was similarly restored as shown by immunocytochemistry and western blotting. Size bars, 100 μm. ( e , f ) Inhibition of classical PKC activity by treatment with Go6976 rescued mRNA expression of additional myogenic genes, including acetylcholine receptor (AchR) and Caveolin 3 (Cav3). The data represent the average of three independent experiments each run in triplicate ±standard deviation. The values from the subconfluent (Subconf) samples were set to 1. The P -values represent two-tailed t -tests for differences between samples indicated. ( g ) PKC phosphorylated recombinant FLAG-tagged Brg1 as shown by 32 P autoradiography. Calcineurin addition inhibited Brg1 phosphorylation by PKC. Quantified data represent the average of three independent experiments ±standard deviation. Two-tailed t -tests showed a significant increase in phosphorylation when Brg1 was treated with PKC, and this phosphorylation decreased when calcineurin was added. A western showing equal loading of FLAG-Brg1 is displayed below the autoradiograph. Full size image We next sought to determine whether repression of myogenesis by PKC is mediated through Brg1. This idea was supported by the fact that PKC was able to phosphorylate purified recombinant Brg1 in-vitro , and this phosphorylation was inhibited in a dose-dependent manner by the addition of purified calcineurin ( Fig. 2g ). There are three classical PKCs known to be inhibited by the drug Go6976: PKCα, PKCβ, which has two splice variants, PKCβI and PKCβII, and PKCγ [31] . All require both a phospholipid ligand, usually diacylglycerol (DAG), and increased calcium concentrations for activity [32] . The proximity ligation assay [33] was used to examine interactions between PKC isoforms and Brg1 ( Fig. 3a–d ). This assay is advantageous because it shows protein–protein interactions in their native context and alleviates the problem of ligand removal during extraction. We identified interactions between Brg1 and PKCβI when cells were sub-confluent ( Fig. 3b–d ). This is notable because it suggests that the interaction between PKCβI and Brg1 exists before the differentiation-induced activation of myogenic gene expression, which is a Brg1-dependent process. The PKCβI interaction with Brg1 is consistent with the fact that we could readily detect PKCβI in the nucleus ( Supplementary Fig. 4b ), while PKCα staining was cytoplasmic ( Supplementary Fig. 4c ). PKCγ was also found in the nucleus ( Supplementary Fig. 4d ), despite its lack of interaction with Brg1. Two different short hairpin RNAs (shRNAs) that knock down PKCβ protein levels in C2C12 cells ( Supplementary Fig. 5a ) partially restored both myogenin and MyHC ( Supplementary Fig. 5b ) expression in the presence of FK506, complementing the PKC inhibitor studies and further demonstrating that in the absence of PKCβ activity, the need for calcineurin activity was reduced. 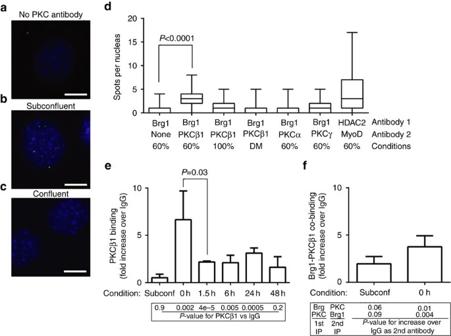Figure 3: PKCβ interacts with Brg1 and blocks differentiation. (a–d) Proximity ligation assay (PLA) was used to detectin-situinteractions between Brg1 and PKC. Representative photomicrographs showing PLA signal (green) and 4,6-diamidino-2-phenylindole staining (blue) are shown of no-PKC antibody controls (a), subconfluent cells with visible nuclear spots (b) and confluent cells (c). The number of nuclear spots was quantified by counting the number of spots per nucleus in 50 nuclei per sample in two independent experiments. Size bars, 5 μm. (d) A statistically significant difference (P<0.0001; Mann–Whitney test, uncorrectedP-value) in the number of signals per nucleus for Brg1 and PKCβI in subconfluent cells was observed when compared with Brg1 antibody alone. Interaction between HDAC2 and MyoD52,53,54was included as a positive control. (e) PKCβI bound to the myogenin promoter in C2C12 cells at the onset of differentiation, but binding decreased as differentiation proceeded (P=0.03; two-tailed unpairedt-test). TheP-values listed below the graph represent one-tailed paired ratiot-tests to test for a significant increase in pulldown compared with IgG in the same experiment. (f) Co-binding of Brg1 and PKCβI occurs as cells became confluent as shown by reciprocal re-ChIPs. The graph represents the values from the Brg1 followed by PKCβI immunoprecipitations. TheP-values shown below the graph represent the results of one-tailed, paired ratiot-tests comparing the control serial pulldown where IgG was substituted for the second antibody. Data ine,frepresent the average from three to six independent experiments each run in duplicate ±s.d. Figure 3: PKCβ interacts with Brg1 and blocks differentiation. ( a – d ) Proximity ligation assay (PLA) was used to detect in-situ interactions between Brg1 and PKC. Representative photomicrographs showing PLA signal (green) and 4,6-diamidino-2-phenylindole staining (blue) are shown of no-PKC antibody controls ( a ), subconfluent cells with visible nuclear spots ( b ) and confluent cells ( c ). The number of nuclear spots was quantified by counting the number of spots per nucleus in 50 nuclei per sample in two independent experiments. Size bars, 5 μm. ( d ) A statistically significant difference ( P <0.0001; Mann–Whitney test, uncorrected P -value) in the number of signals per nucleus for Brg1 and PKCβI in subconfluent cells was observed when compared with Brg1 antibody alone. Interaction between HDAC2 and MyoD [52] , [53] , [54] was included as a positive control. ( e ) PKCβI bound to the myogenin promoter in C2C12 cells at the onset of differentiation, but binding decreased as differentiation proceeded ( P =0.03; two-tailed unpaired t -test). The P -values listed below the graph represent one-tailed paired ratio t -tests to test for a significant increase in pulldown compared with IgG in the same experiment. ( f ) Co-binding of Brg1 and PKCβI occurs as cells became confluent as shown by reciprocal re-ChIPs. The graph represents the values from the Brg1 followed by PKCβI immunoprecipitations. The P -values shown below the graph represent the results of one-tailed, paired ratio t -tests comparing the control serial pulldown where IgG was substituted for the second antibody. Data in e , f represent the average from three to six independent experiments each run in duplicate ±s.d. Full size image We next sought to determine whether PKC/Brg1 interactions and the potential negative effect of PKC phosphorylation on Brg1 could be observed at chromatin. PKCβI was not bound to the myogenin promoter in proliferating cells, but was bound to the myogenin promoter when cells became confluent ( Fig. 3d ), with a notable decrease after differentiation began (1.5 h; Fig. 3e ). This binding is consistent with PKCβI being brought to the promoter along with Brg1 recruitment in confluent cells ( Fig. 1b ), and was confirmed by sequential ChIP experiments ( Fig. 3f ). Taken together, these results suggest that Brg1 is associated with PKCβI when recruited to the myogenin promoter in confluent cells but PKCβI binding is quickly reduced, possibly due to the activity of calcineurin, which is already present at the promoter ( Fig. 1d ). Failure to detect co-binding of PKCβI and calcineurin to the same chromatin fragments by re-ChIP ( Supplementary Fig. 5c ) suggests mutually exclusive binding or that any possible intermediate structure containing PKCβI, Brg1 and calcineurin is quickly resolved with the loss of PKCβI from the promoter. When combined with the observation that Brg1/PKCβI interaction is reduced in confluent cells ( Fig. 3a–d ), these data support the idea that while overall interaction between Brg1 and PKCβI is reduced as Brg1 is brought to the promoter, sufficient interaction remains to bring PKCβI to the promoter, where the interacting proteins can still be detected by the very sensitive re-ChIP assay. Promoter binding by PKCβI may play a role in preventing Brg1 from stably binding until signalling through calcineurin occurs. PKC target residues flank the Brg1 bromo domain To address the possible function of PKC phosphorylation on Brg1, we identified Brg1 residues that could be phosphorylated by PKC. An initial search for functional PKC sites utilized glutathione S -transferase (GST) fusions across the length of Brg1 ( Supplementary Fig. 6a ) and identified two C-terminal fragments (#5, #6) flanking or containing the bromodomain that could be phosphorylated by PKC in-vitro ( Supplementary Fig. 6b–d ). Mutations of these two fragments identified amino acids 1,620 ( Supplementary Fig. 6e ), 1,617 ( Supplementary Fig. 6f ), 1,409/10 ( Supplementary Fig. 6g ) and multiple amino acids between 1,417 and 1,430 ( Supplementary Fig. 6g ) as targets of PKC phosphorylation. Mutation of an independent fragment comprising fragments #5 and #6 and the carboxyl terminus confirmed these results; mutation of 1,409/10 and 1,617/20 reduced the phosphorylation of this fragment ( Fig. 4a ), and deletion of the multiple serine/threonine containing region 1,417–1,430 further reduced phosphorylation ( Fig. 4a ). 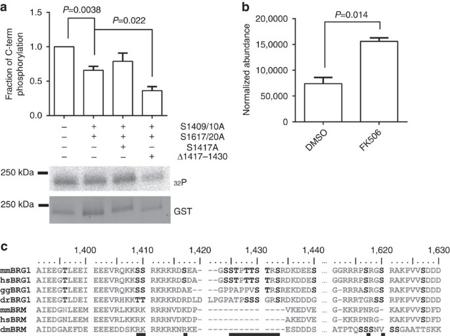Figure 4: Amino acids (aa) flanking the Bromo domain of Brg1 are phosphorylated by PKC. (a) Mutation of aa 1,409/1,410 and aa 1,617/1,620 to alanine significantly reduced the phosphorylation of a C-terminal Brg1 fragment (aa 1,360–1,647) by PKC. Further deletion of aa 1,417–1,430 reduced phosphorylation compared with mutation of aa 1,409/10 and aa 1,617/20. The data represent the average of three independent experiments ±s.d. The values for the C-terminal fragment (lane 1) were set to 1. A representative image of reactions that were run on SDS–PAGE, transferred to PVDF membrane, exposed to a Phosphorimager and subsequently developed as a western blot to visualize the GST fusion proteins, is shown. (b) A phospho-peptide containing aa 1,417-1,430 was identified by mass spectrometry and quantified from the extracted ion chromatogram. The graph shows that the normalized abundance of the peptide was increased in the absence of calcineurin signalling.P-values ina,bare the result of two-tailedt-tests. (c) Alignment of the PKC phosphorylated region of Brg1 between mouse (mm), human (hs), chicken (gg), zebrafish (dr) andDrosophila(dm) Brg1 and Brm showed a number of serine and threonine residues that are conserved among Brg1 homologues, but not with the paralogous regions of Brm. Black bars beneath the alignment show regions identified as phosphorylated by PKC. Figure 4: Amino acids (aa) flanking the Bromo domain of Brg1 are phosphorylated by PKC. ( a ) Mutation of aa 1,409/1,410 and aa 1,617/1,620 to alanine significantly reduced the phosphorylation of a C-terminal Brg1 fragment (aa 1,360–1,647) by PKC. Further deletion of aa 1,417–1,430 reduced phosphorylation compared with mutation of aa 1,409/10 and aa 1,617/20. The data represent the average of three independent experiments ±s.d. The values for the C-terminal fragment (lane 1) were set to 1. A representative image of reactions that were run on SDS–PAGE, transferred to PVDF membrane, exposed to a Phosphorimager and subsequently developed as a western blot to visualize the GST fusion proteins, is shown. ( b ) A phospho-peptide containing aa 1,417-1,430 was identified by mass spectrometry and quantified from the extracted ion chromatogram. The graph shows that the normalized abundance of the peptide was increased in the absence of calcineurin signalling. P -values in a , b are the result of two-tailed t -tests. ( c ) Alignment of the PKC phosphorylated region of Brg1 between mouse (mm), human (hs), chicken (gg), zebrafish (dr) and Drosophila (dm) Brg1 and Brm showed a number of serine and threonine residues that are conserved among Brg1 homologues, but not with the paralogous regions of Brm. Black bars beneath the alignment show regions identified as phosphorylated by PKC. Full size image We attempted to detect phosphorylation of these peptides directly using TiO 2 phospho-peptide enrichment followed by detection by MS. A phosphopeptide was identified corresponding to the 1,417–1,430 region ( Supplementary Fig. 7a–c ). The MS/MS spectrum indicates that this peptide is most likely phosphorylated on Serine 1,421 or 1,422, however, it should be noted that the Mascot Delta Ion Score [34] is 0, indicating it is not possible to distinguish between the multiple potential phosphorylation sites on this peptide. The retention and mass coordinates of the peptide were used to identify the location of the phosphopeptide in the ion chromatograph of total Brg1 samples from FK506- or DMSO-treated cells. The peaks were quantified and a significant difference was observed between FK506- and DMSO-treated cells ( Fig. 4b ), indicating hyperphosphorylation of this fragment in calcineurin-inhibited cells. The identification of Brg1 phosphopeptides that include amino acids between 1,410 and 1,430 in the PhosphoSitePlus database [35] provides additional evidence that phosphorylation of this region occurs in a number of systems and may have broad implications for control of Brg1 function. Alignment of Brg1 and the closely related Brm enzyme reveal that these sites are highly conserved in Brg1 from fish to humans, but are not present in Brm ( Fig. 4c ). This suggests that the ability to be phosphorylated by PKC is a trait unique to Brg1. Given the essential role of Brg1 in differentiation and the dispensability of Brm for mouse development and viability [14] , PKC regulation of Brg1 may be one of the important functional differences between these two otherwise similar proteins. The identification of phosphorylation sites in this region implies a regulatory function for this region, either through association of Brg1 with other factors or through modulation of Brg1 activity. To test the significance of Brg1 phosphorylation in myogenesis, we sought to replace endogenous Brg1 with full-length, Yellow Fluorescent Protein (YFP)-tagged, wild-type Brg1 (WT-Brg1) or the C-terminal phosphomimetic (SE-Brg1) or non-phosphorylatable (SA-Brg1) mutants described above ( Supplementary Fig. 8a ). We were unable to generate Brg1-deficient C2C12 cells; instead we isolated satellite cells from mice homozygous for a conditional Brg1 allele [11] that could be removed by Cre recombinase. These cells were propagated in culture and infected with a mCherry-expressing retrovirus, in which exogenous, YFP-tagged Brg1 would replace mCherry only after recombination of the integrated retroviral vector by Cre ( Supplementary Fig. 8b ). Thus, exogenous, YFP-labelled Brg1 would stably replace the endogenous protein in the presence of Cre recombinase ( Supplementary Fig. 8c ). Previous studies utilized Cyclosporin A (CsA) as an effective inhibitor of calcineurin activity and differentiation in primary human myoblasts [36] and in in-vivo muscle regeneration in mouse [36] . We found that in primary satellite cell cultures, inhibition of calcineurin through administration of CsA resulted in inhibition of myotube formation ( Supplementary Fig. 8d ). Expression of CAIN also inhibited myogenesis in primary myoblasts, with a similar reduction in myotube length and nuclei content, but without loss of myogenin or MyHC expression ( Supplementary Fig. 8e ). Unlike CsA-treated cells, however, CAIN-expressing cells exhibited increased cell death upon differentiation. Addition of Go6976 resulted in accelerated differentiation ( Supplementary Fig. 8f ). These results suggest that PKC activity blocks myoblast fusion and reinforce the idea that PKC opposes calcineurin function in primary satellite cell-derived myoblast cultures. For each form of Brg1, wild type (WT-Brg1), phosphomimetic (SE-Brg1) and non-phosphorylatable (SA-Brg1), we generated mCherry-positive clones that differentiated well in the absence of Ad-Cre and that expressed YFP in the nuclei of >95% of cells when exposed to Ad-Cre ( Supplementary Fig. 8g ). Cre-induced replacement of endogenous Brg1 with WT-Brg1 did not affect myogenesis ( Fig. 5a , top left) compared with untreated controls ( Supplementary Fig. 8h ). Furthermore, the number of nuclei per myotube did not differ between myotubes from Cre-treated and untreated cultures ( Fig. 5b ). Cells expressing WT-Brg1 were also sensitive to CsA treatment, which resulted in the formation of myotubes that failed to elongate ( Fig. 5a , top right, arrowheads), and had significantly fewer nuclei ( Fig. 5b ). This phenotype was mimicked by replacement of endogenous Brg1 with SE-Brg1. Before administration of Ad-Cre, SE-Brg1 clones differentiated normally as judged by the number of nuclei per myotube ( Fig. 5b , middle), whereas Cre-induced replacement of Brg1 resulted in unfused cells, shortened, rounded myotubes ( Fig. 5a , middle-left, arrowheads), and a significant reduction in the number of nuclei per myotube ( Fig. 5b ). These results were not further affected by the presence of CsA ( Fig. 5a , middle). Replacement with the non-phosphorylatable SA-Brg1 did not significantly affect myotube formation ( Fig. 5a , bottom), or the number of nuclei per myotube ( Fig. 5b ). Furthermore, treatment of these cells with CsA neither impaired myogenesis ( Fig. 5a , bottom-right) nor reduced nuclei content ( Fig. 5b ), showing that the effect of CsA is mediated by hyper-phosphorylation of Brg1. Similar results were found in myoblasts expressing the CAIN inhibitor ( Supplementary Fig. 8i ). Cells expressing WT-Brg1 or SA-Brg1 in the absence of CAIN differentiated and formed myotubes with similar numbers of nuclei per myotube. Cells expressing WT-Brg1 responded to CAIN expression with a decrease in myotube length and number of nuclei per myotube compared with cells infected with empty vector. In contrast, cells expressing SA-Brg1 formed longer myotubes with more nuclei per myotube, as expected. 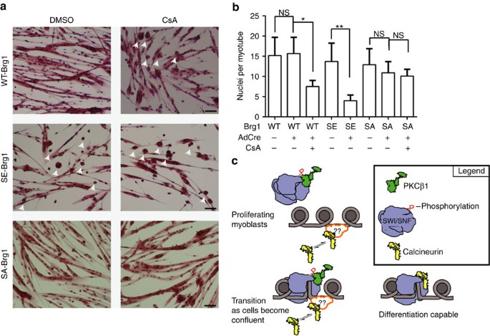Figure 5: PKC phosphorylation of Brg1 controls differentiation. (a) H & E staining of primary myoblasts differentiated for 4 days shows that addition of Ad-Cre and DMSO (left column) resulted in shortened myotubes only in the cells where endogenous Brg1 was replaced with phosphomimetic Brg1 (SE-Brg1; middle row, arrowheads). When differentiated in the presence of CsA (right column), Ad-Cre-treated cells expressing wild type or SE-Brg1 differentiated into shortened myotubes (arrowheads) with fewer nuclei than their untreated counterparts, whereas cells expressing non-phosphorylatable Brg1 (SA-Brg1) were resistant to the effects of CsA and showed elongated myotubes, with similar nuclear content to the untreated cells. Size bars, 100 μm. (b) Summary of median nuclei number across multiple experiments and clones. WT-Brg1 data are the summary of one clone and three independent trials, SE-Brg1 is summary of two clones with three independent trials each, and SA-Brg1 is three clones with two independent trials each. 50 or more myotubes were counted in each sample of each trial. *P=0.034, **P=0.0018 by two-tailedt-test; NS, not significant. (c) A model showing the role of calcium-dependent phosphorylation in regulating chromatin remodelling. In sub-confluent, proliferating myoblasts, calcineurin is weakly bound to chromatin, probably through interaction with an as yet unknown factor, whereas SWI/SNF enzyme is bound by PKCβI, not in association with the chromosome. Once differentiation begins, SWI/SNF begins to be associated with the chromatin along with PKCβI. Within 1.5 h, there is a significant decrease in PKCβI association with the promoter, and a significant increase in calcineurin and Brg1 association with the promoter. This structure is stable and results in chromatin remodelling, leading to gene expression. Figure 5: PKC phosphorylation of Brg1 controls differentiation. ( a ) H & E staining of primary myoblasts differentiated for 4 days shows that addition of Ad-Cre and DMSO (left column) resulted in shortened myotubes only in the cells where endogenous Brg1 was replaced with phosphomimetic Brg1 (SE-Brg1; middle row, arrowheads). When differentiated in the presence of CsA (right column), Ad-Cre-treated cells expressing wild type or SE-Brg1 differentiated into shortened myotubes (arrowheads) with fewer nuclei than their untreated counterparts, whereas cells expressing non-phosphorylatable Brg1 (SA-Brg1) were resistant to the effects of CsA and showed elongated myotubes, with similar nuclear content to the untreated cells. Size bars, 100 μm. ( b ) Summary of median nuclei number across multiple experiments and clones. WT-Brg1 data are the summary of one clone and three independent trials, SE-Brg1 is summary of two clones with three independent trials each, and SA-Brg1 is three clones with two independent trials each. 50 or more myotubes were counted in each sample of each trial. * P =0.034, ** P =0.0018 by two-tailed t -test; NS, not significant. ( c ) A model showing the role of calcium-dependent phosphorylation in regulating chromatin remodelling. In sub-confluent, proliferating myoblasts, calcineurin is weakly bound to chromatin, probably through interaction with an as yet unknown factor, whereas SWI/SNF enzyme is bound by PKCβI, not in association with the chromosome. Once differentiation begins, SWI/SNF begins to be associated with the chromatin along with PKCβI. Within 1.5 h, there is a significant decrease in PKCβI association with the promoter, and a significant increase in calcineurin and Brg1 association with the promoter. This structure is stable and results in chromatin remodelling, leading to gene expression. Full size image A model for PKCβI/calcineurin function Our results identify PKCβ as a regulator of myogenesis that functions in opposition to calcineurin and indicate that PKC and calcineurin act by modifying Brg1. Calcium signalling is common to many differentiation pathways as well as a variety of cellular functions, including cell cycling. [37] It is not surprising, therefore, that mechanisms exist to differentiate calcium signalling events that relate to a specific function. Our data provide evidence for a model in which regulation of SWI/SNF function is passed from one calcium-sensitive pathway to another through modification of the enzymatic subunit Brg1 ( Fig. 5c ). In subconfluent, proliferating myoblasts, Brg1 is bound by PKCβI ( Fig. 3b,d ), but is not bound to chromatin ( Fig. 3e ). Meanwhile, calcineurin is in contact with the promoter, but is not yet strongly bound ( Fig. 1d ). Because there are no reports of calcineurin having independent DNA-binding activity, it is presumed to bind through an as yet unknown partner. Once cells become confluent and begin to differentiate, SWI/SNF is recruited to the myogenin promoter ( Fig. 1b ) with PKCβI ( Fig. 3e ; 0 h). Whether there is a short-lived intermediary structure or whether Brg1/PKCβI can only bind to promoters unoccupied by calcineurin remains to be determined, but within the first 1.5 h, the promoter is predominantly occupied by Brg1/calcineurin. We propose that the ability of calcineurin to dephosphorylate Brg1 promotes its positive activity in promoting differentiation. The nature of the switch between the inhibitory effects of PKCβI and its reversal by calcineurin remains to be elucidated. One possibility is the presence of DAG, the PKC ligand, in the nucleus accounts for the activity of PKCβI, which gives way to calcineurin due to decreases in nuclear DAG. DAG is derived from phospholipids and is normally considered a cell membrane component, but it is also found in a variety of nuclear compartments including splicing speckles and chromatin [38] . Furthermore, nuclear forms of the enzymes responsible for DAG production, such as phospholipase C [39] , [40] , and inactivation, such as DAG kinase [41] , are found in the nucleus and have been shown to impact differentiation of muscle cells. In addition to potential changes in DAG signalling, the calcium signal itself may contribute to differential activation of calcineurin and PKCβ. The existence of both of these proteins in the nucleus suggests that nuclear calcium content may control transcriptional activity. The existence of calcium transients in the nucleus has been confirmed by the use of nuclear localized calcium reporters [42] , [43] , but the source of the calcium influx has not yet been determined. Differences in spatial pattern, duration or amplitude of the signal may all play a role in differentially activating calcineurin and PKCβ. We suggest that Brg1 acts as a nexus through which opposing calcium-dependent signals controlling differentiation exert their effects. The identification of Brg1, which provides catalytic activity to the SWI/SNF enzyme and is required for most tissue differentiation events, as a target of multiple signal transduction pathways suggests a common mechanism by which these distinct pathways are integrated and balanced to exert control over the expression of differentiation-specific genes. The regulation of Brg1 function is potentially complemented by a more specific level of SWI/SNF enzyme regulation by signalling pathways, as the cardiac- and skeletal muscle-specific SWI/SNF subunit, Baf60c, has also been identified as a key target of the p38 MAP kinase pathway during differentiation [8] , [16] . Thus, signal transduction-mediated regulation of the function of the more ubiquitous catalytic subunit may be further refined by additional signal transduction-mediated control of the function of a tissue-specific enzyme subunit. The importance and specificity of this regulatory mechanism are highlighted by the identification of residues unique to Brg1 that are not found in its closely related but dispensable homologue, Brm. Thus, the ability to be targeted by signal transduction pathways may be an important functional difference between these two similar ATPases. In conclusion, the data support the idea that Brg1 and the SWI/SNF complex as a whole, is a critical target for integrating distinct signalling cues during cellular differentiation. Generation of plasmids GST–Brg1 fusions were made by amplifying fragments of Brg1 from pBluescript Flag-Brg1 (ref. 44 ) using the primers listed in Supplementary Table 2 and cloning them into pGEX-2T. Mutations of fragments #5, #6, and the C-term fragment were generated using the Quickchange Lightning Multi-site Directed Mutagenesis kit (Agilent) using primers listed in Supplementary Table 2 . Mutations were verified by sequencing. To make full-length mutant Brg1, the ClaI fragment was excised from pBluescript Flag-Brg1 (ref. 44 ), blunted, and cloned into the EcoRV site of pCR3.1 (Invitrogen). The Bss HI site in the pCR3.1 vector was then removed by excising the fragment containing the neomycin-resistant gene using Stu I and Bst BI. The mutated C-term fragments were then cloned into full-length pCR3.1-Brg1 using Bss HI and Sal I restriction sites. The wild-type and mutant Brg1 sequences were fused to YFP by cutting the Nhe I- Bam HI fragment out of the EYFP-c1-Brg1 (ref. 45 ; gift of Gordon Hager), which contained YFP fused to the N-terminus of Brg1, and cloning it into Age I- Bam HI-digested pCR3.1-Brg1 for each Brg1 sequence. The inducible pBabe vector was generated by amplifying the LoxP-mCherry sequence using primers listed in Supplementary Table 2 from the vector hsp70l-loxP-mCherry-STOP-loxP-H2B-GFP_cryaa-cerulean [46] , digesting with Eco RI/ Bgl II, and ligating it and an additional LoxP site with a short polylinker generated by two overlapping oligonucleotides ( Supplementary Table 2 ) into the Eco RI- Sal I site of pBabe-puro using a three-way ligation. The resulting vector was cut with Age I and Pme I as was the pCR3.1-YFP-Brg1, and the YFP-Brg1 fragment was ligated in. pBABE FLAG-CAIN was created using primers containing the FLAG sequence and homology to mouse CAIN ( Supplementary Table 2 ) to amplify CAIN from the BF10 plasmid [20] (gift of Grace Pavlath) and cloned into the Sal I and Eco RI sites of pBabe-puro, which was used for C2C12 experiments, or pBabe-blastocydin, which was used for primary myoblast experiments. shRNA sequences that targeted both isoforms of PKCβ are listed in Supplementary Table 2 . The sequences were cloned into pENTR/pTER+ (ref. 47 ) and then introduced to pLenti x2 DEST (puro) [47] via recombination. Recombination was performed using the LR clonase mix according to the manufacturer’s instructions (Invitrogen). Cell culture C2C12 cells were purchased from American Type Culture Collection (CRL-1772). Differentiation of C2C12 cells was initiated by plating 4 × 10 4 or 1 × 10 5 cells in 12- or 24-well plates, respectively, in DMEM media containing 10% fetal bovine serum. After 48 h, cells reached confluence, the media was changed to DMEM containing 2% horse serum, and the cells were allowed to differentiate for 48 h, except where noted. FK-506 (Cayman Chemical) was added to the culture at 24 h after plating and included in the differentiation media at 500 nM. Go6976 (CalBiochem) was added to the differentiation media at a concentration of 500 nM. Retrovirus was produced as previously described [48] . Briefly, 10 μg of DNA for each construct were transfected into Bosc23 cells [49] using Lipofectamine 2,000 (Invitrogen). The viral supernatant was collected after 48 h and filtered through a 0.45μm syringe filter (Millipore). C2C12 cells were infected with retrovirus in the presence of 8 μg ml −1 polybrene and selected for 2 days with 1 μg ml −1 puromycin (Invitrogen). Surviving cells were then plated and differentiated as described above. shRNA-expressing lentivirus was produced as described [47] . Briefly, the lentiviral construct DNA was co-transfected with the pLP1, pLP2 and pVSVG packaging vectors into 293T cells (American Type Culture Collection; CRL-3216) with Lipofectamine 2,000 reagent (Invitrogen). The viral supernatant was collected after 48 h and filtered through a 0.45-μm syringe filter (Millipore). C2C12 cells were infected with lentivirus and selected for 2 days with 1 μg ml −1 puromycin. Surviving cells were then plated and differentiated in the presence or absence of FK506 as described above. Mice were housed in the animal care facility at the University of Massachusetts Medical School (Worcester, MA, USA) in accordance with the Institutional Animal Care and Use Committee guidelines. Mouse satellite cells were purified from total leg muscle from 3- to 6–week-old male and female Brg1 conditional mice [11] by differential plating following Purcol sedimentation as previously described [50] . Briefly, excised muscle tissue was rinsed with Hank’s Balanced Salt Solution (HBSS; Life Technologies), sliced into small pieces and incubated with 0.1% Pronase in HBSS at 37 °C for 60 min. The cell suspension was filtered using a 100-μm cell sieve and resuspended in 3 ml of growth media containing a 1:1 mix of DMEM and F-10 supplemented with 20% fetal bovine serum, 2% Chick Embryo Extract (Sera Laboratories) and 25 ng ml −1 recombinant basic FGF (Millipore). Cells were filtered again using a 40-μm cell sieve and centrifuged at 1,000 g for 1 min at room temperature. The cells were placed in the top of the Percoll gradient (35 and 70%) and centrifuged 20 min at 1,850 g at room temperature. The population of myoblasts contained in the lower interface of the 70% Percoll fraction was washed with HBSS, centrifuged 5 min at 1,000 g , and resuspended in growth media for plating. Isolated cells were grown and differentiated on plates coated overnight in 0.02% collagen (Advanced BioMatrix). Cells were differentiated in 2% horse serum for up to 4 days. For retrovirus infection, retrovirus was concentrated using Retro-X concentrator (Clontech) and cells were infected in 8 μg ml −1 polybrene at a multiplicity of infection (MOI)<1 and selected with 1 μg ml −1 puromycin. For clone isolation, after 2 days of puromycin selection, cells were replated at low density and allowed to grow for 1 week. mCherry-expressing colonies were picked using cloning rings and transferred to collagen-coated wells of 96-well plates. Media were changed every other day, and cells were transferred to a new collagen-coated well every 5 days, choosing a dish size appropriate for the number of cells. Once there were sufficient cells to reach 50% confluence on a 60-mm dish, cells were tested for differentiation and transgene expression. To make CAIN-expressing cells and pBABE controls, retrovirus was produced as described above and clones were infected as described. After 24 h of infection, cells were selected for 4 days using 4 μg ml −1 blastocidin, then treated with adenovirus as described below. Adenovirus for expression of Cre-recombinase (Ad-Cre; University of Iowa Gene Transfer Vector Core) [51] was administered at an MOI of 50. Clones were chosen based on >99% of the cells expressing YFP-Brg1 in Cre-treated cells and a fusion index near 100% in cells not treated with Cre recombinase. For differentiation, 2 days following Ad-Cre treatment, cells were re-plated such that they were 50% confluent at the start of differentiation. CsA (Cell Signaling) was added at a concentration of 2 μM 2 days before induction with CsA-containing differentiation media. Go6976 was added at a concentration of 500 nM 24 h after plating. Immunocytochemistry Cells grown on 12- or 24-well plates were stained with anti-myosin heavy chain (MF20) or anti-myogenin (F5D) antibodies obtained as hybridoma supernatants from the Developmental Studies Hybridoma Bank. After differentiation, cells were fixed in formalin, then incubated overnight with hybridoma supernatant at a 1:100 dilution along with 5% horse serum, 0.2% Triton X-100 in 1 × PBS. Secondary antibody binding and HRP staining were performed with the ABC anti-mouse kit (Vector Labs) according to the manufacturer’s protocol. Immunofluorescence for MHC and myogenin was performed as described above, except that the antibodies were used at a 1:10 dilution, and secondary detection was accomplished using an Alexa-Fluor 488-labelled secondary antibody (1:500; Invitrogen). Cells were counterstained with 4,6-diamidino-2-phenylindole. Mouse monoclonal antibodies against PKCα, PKCβI and PKCγ (H7, E3 and D4, respectively) were obtained from Santa Cruz and used at a 1:100 dilution. For counting myogenin-positive and 4,6-diamidino-2-phenylindole-stained nuclei, five separate fields were imaged for each of three data points per condition, and counting was done automatically using CellProfiler ( http://www.cellprofiler.org/ ). Proximity ligation assay was performed using DuoLink Mouse Plus and Rabbit Minus secondary antibodies and staining kit (O-Link Biosciences) using antibodies against Brg1 (1:100 dilution; H-88, Santa Cruz), and PKCβI (1:100 dilution; sc-8049, Santa Cruz), following the manufacturer’s instructions. As a control, mouse anti-MyoD (1:100 dilution; Abcam) and rabbit anti-HDAC2 (1:100 dilution; Zymed) were used to quantify the MyoD/HDAC2 interaction [52] , [53] , [54] . Western blots and co-IP Scraped cells were washed with PBS and solubilized in RIPA buffer (10 mM piperazine-N,N′-bis(2-ethanesulfonic acid), pH 7.4, 150 mM NaCl, 2 mM EDTA, 1% Triton X-100, 0.5% sodium deoxycholate and 10% glycerol) containing Complete Mini protease inhibitor (Roche). Equivalent amounts of each extract were boiled in SDS-sample buffer and subjected to SDS–polyacrylamide gel electrophoresis. The resolved proteins were transferred to a polyvinylidene difluoride (PVDF) membrane (Bio-Rad) and incubated with antibodies against proteins of interest, followed by species-appropriate peroxidase-conjugated antibodies (1:1,000 dilution; Pierce) and chemiluminescent detection as directed by the manufacturer (ECL PLUS; GE Healthcare). Antibodies used included myosin heavy chain (1:100 dilution; Developmental Studies Hybridoma Bank), GST (1:500 dilution; Invitrogen), FLAG (1:1,000 dilution [25] ), PKCβI (1:1,000 dilution; sc-8049, Santa Cruz) and mouse anti-GAPDH-Peroxidase conjugated (1:1,000 dilution; G9295, Sigma-Aldrich). For the co-IP experiments, C2C12 cells were differentiated in media containing 2% horse serum for 24 h. Monolayers were washed three times in PBS and resuspended in lysis buffer (25 mM Tris, pH 7.5, 1 mM CaCl2, 150 mM NaCl, 0.5% NP40) and homogenized by eight strokes using a glass dounce homogenizer. Cell lysates were incubated overnight at 4 °C in an orbital shaker with the following antibodies: Brg1 antiserum [55] (10 μl), anti-Baf155 (15 μg; Santa Cruz), anti-Calcineurin (10 μg; Cell Signaling Technology), anti-mouse IgG (15 μg; Santa Cruz). Samples were then incubated for 2 h at 4 °C with protein A sepharose (Invitrogen). Samples were washed three times with buffer containing 25 mM Tris, pH 7.5, 1 mM CaCl 2 , 300 mM NaCl, 0.5% NP40. Immunoprecipitated complexes were eluted in Laemmli Buffer by boiling the samples for 10 min and were analysed by western blot as indicated above. Uncropped images are presented in Supplementary Fig. 9 . Restriction enzyme accessibility and ligation-mediated PCR Restriction enzyme accessibility assay was carried out as described [25] , [56] . Briefly, cells were washed in PBS and nuclei isolated by incubation in lysis buffer (10 mM PIPES, pH 8, 85 mM KCl, 1 mM CaCl 2 , 5% sucrose, 0.5% NP40, plus protease inhibitors added immediately before use, including 1 μg ml −1 leupeptin and 1 mM phenylmethylsulphonyl fluoride) followed by centrifugation at 300 g for 2 min at 4 °C. Nuclei were then incubated with PvuII (NEB) in the appropriate restriction buffer. Cutting was assayed by ligating a linker fragment, followed by SYBR green quantitative PCR (ABI) using primers against the linker and the PvuII site in the myogenin promoter [25] , [56] . ChIP assays ChIP assays using cultured C2C12 cells were performed as described [57] , [58] . Briefly, cells were cross-linked with 1% formaldehyde and lysed in buffer containing 1% SDS, 10 mM EDTA, pH 8, and 50 mM Tris-HCl, pH 8, with Complete Mini-Protease inhibitor (Roche). After sonication, chromatin was pre-cleared for 1 h with protein A-agarose beads blocked with salmon sperm DNA (Millipore). Cell lysates were incubated overnight with antibodies against Pan-Calcineurin A (10 μg; Cell Signaling Technology, 2,614) or PKCβI (10 μg; Santa Cruz, sc-8,049), polyclonal rabbit antisera against Brg1 (ref. 55 ; 10 μl) or normal rabbit IgG (15 μg; Santa Cruz, sc-3888) and immunoprecipitated material was collected with Magna ChIP Protein A+G Magnetic Beads (Millipore). Cross-linking was reversed, and DNA was purified using ChIP DNA Clean & Concentrator Columns (Zymo Research). Quantitative PCR utilized Fast SYBR green master mix on the ABI StepOne Plus Sequence Detection System. Quantification was performed using the comparative Ct method to obtain the percent of total input DNA pulled down by each antibody. The value for each antibody was divided by the amount precipitated by the amount of DNA precipitated by normal IgG in the same experiment. To ascertain the statistical significance of binding by the studied factors, amounts of DNA pulled down by the antibody was paired with the IgG control that was performed alongside the tested antibody, and three to six independent results were pooled for a pairwise Student’s t -test. To test for significant changes in binding, replicate values of the antibody divided by the IgG control were subjected to a Student’s t -test. Re-ChIP, or sequential ChIP, experiments were performed as described [59] . Briefly, after incubating the samples with the first antibody of interest and collecting immunoprecipitated material with magnetic beads, the samples were incubated with an equal volume of 10 mM dithiothreitol for 30 min at 37 °C. The supernatant was used for the second immunoprecipitation by adding the second antibody of interest and incubating as with the first antibody. IgG substituted as the second antibody as a control. Quantification and statistical tests were done as described above. In-vitro phosphorylation assays Baculovirus produced recombinant FLAG-tagged BRG1 was purified [10] . Purified recombinant PKC and calcineurin were obtained from Sigma, and PKC activator was obtained from Millipore. PKC was incubated for 30 min with equal amounts of rBRG1 in the presence of PKC activator that had been sonicated for 1 min and 25 μM ATP containing 32 P-labelled ATP. After incubation, samples were mixed with loading buffer and electrophoresed, then transferred to PVDF membrane (Bio-Rad). After exposure to a phosphorimaging plate, the membrane was developed using anti-FLAG antisera [25] at a 1:1,000 dilution. GST–Brg1 fragments were produced in BL-21 E. coli by induction with 0.5 mM isopropyl-β- D -thiogalactoside for 4 h. Bacterial pellets were sonicated and bound to GST-agarose beads (Pierce) in 1 × PBS with protease inhibitors (Roche), followed by three washes in 1 × PBS and elution with 20 mM reduced glutathione in 50 mM Tris, pH 8.1. For each mutant, 100 ng of purified protein was added to the PKC reaction described above. Owing to the presence of a co-migrating PKC auto-phosphorylation band, the C-terminal fragment ( Supplementary Fig. 3d ) was rebound to GST beads after kinase treatment and washed with three times with 1 × PBS, followed by elution in loading buffer. The reactions were run on an SDS–PAGE gel and transferred to PVDF, which was exposed to a phosphorimaging plate, then developed using an anti-GST antibody (1:500 dilution; Invitrogen). Secondary staining was done using AF546–labelled anti-rabbit antibody (1:1,000 dilution; Invitrogen), and blots were scanned using a Typhoon laser imager (Molecular Dynamics). GST western and phosphorimaging was quantified using ImageQuant (Molecular Dynamics) and the phosphorimage signal was normalized to the GST signal. Uncropped images are presented in Supplementary Fig. 9 . Brg1 purification for MS Brg1 was purified from 15 15 cm plates of C2C12 cells that had been differentiated for 24 h. Cell pellets were sonicated in SDS-lysis buffer (50 mM Tris, pH 8.1, 10 mM EDTA, 1% SDS), then diluted in IP buffer (0.01% SDS, 1.1% Triton X-100, 1.2 mM EDTA, 16.7 mM Tris, pH 8.1, 167 mM NaCl). Brg1 was purified using an antiserum against the N-terminus [25] bound to protein A beads (Millipore), followed by washes in Buffer A (0.1% SDS, 1% Triton X-100, 2 mM EDTA, 20 mM Tris, pH 8.1, 150 mM NaCl), Buffer B (Same as Buffer A, but 500 mM NaCl), Buffer C (0.25 M LiCl, 1% NP-40, 1% sodium deoxycholate, 1 mM EDTA, 10 mM Tris, pH 8.1) and TE (10 mM Tris pH 8.0, 1 mM EDTA). All buffers contained protease and phosphatase inhibitors (Roche). Brg1 was then eluted in SDS-loading buffer, submitted to SDS–PAGE followed by Coomassie staining, and the Brg1 band was cut out of the gel. BSA was run for quantitation. ∼ 800 ng of Brg1 was purified. In gel digestion of Brg1 Gel slices were cut into 1 × 1 mm 2 pieces and placed in 1.5 ml eppendorf tubes with 1 ml of water for 1 h. The water was removed and 50 μl of 250 mM ammonium bicarbonate was added. For reduction, 5 μl of a 45 mM solution of 1,4 dithiothreitol was added, and the samples were incubated at 50 °C for 30 min. The samples were cooled to room temperature and alkylated for 30 min with 5 μl of 100 mM iodoacetamide. The gel slices were washed twice with 1 ml water aliquots. The water was removed, 1 ml of 50:50 (50 mM ammonium bicarbonate/acetonitrile) was placed in each tube, and samples were incubated at room temperature for 1 h. The solution was then removed and 200 μl of acetonitrile was added to each tube, at which point the gels slices turned opaque white. The acetonitrile was removed and gel slices were further dried in a Speed Vac. Gel slices were rehydrated in 50 μl of 2 ng μl −1 trypsin (Sigma) in 0.01% ProteaseMAX Surfactant (Promega)/50 mM ammonium bicarbonate. An additional aliquot of 50 mM ammonium bicarbonate was added to fully submerge the gel slices. Samples were incubated at 37 °C for 21 h. The supernatant of each sample was then removed and placed in a new 1.5-ml eppendorf tube. Gel slices were further dehydrated with 100 μl of 80:20 (acetonitrile/1% formic acid). The extract was combined with the supernatants of each sample. The samples were then dried in a Speed Vac. Isobaric labelling and MS analysis Brg1 purified from either DMSO- or FK506-treated cells was trypsin digested, and each sample was split into two equal aliquots and labelled with a unique iTRAQ label (Invitrogen) following the manufacturer’s instructions. One aliquot from each of the DMSO- or FK506-treated samples was treated for 3 h in 2U shrimp alkaline phosphatase (Promega) plus 2U calf intestine phosphatase (NEB) in CIP Buffer 3 (NEB), whereas the other half of each sample was treated in buffer alone. Samples were then purified using C20 resin, eluted in 80% acetonitrile, 0.1% trifluoroacetic acid (TFA), then dried and resuspended in water. Before analysis, samples were mixed together and were spiked with 100 fmol of pre-digested yeast alcohol dehydrogenase (ALDH) as an internal standard. Gel extracted tryptic peptides were injected using a NanoAquity auto sampler onto a Symmetry C18 trapping cartridge (180 μm i.d. × 2 cm length; Waters, Inc.) at a flow rate of 5 μl min −1 for 3 min. Next, peptides were separated by in-line gradient elution onto a 75 μm i.d. × 10 cm column packed with BEH 130 Stationary phase (Waters), 1.7 μm particle size, at a flow rate of 300 nl min −1 using a linear gradient from 2 to 40% B over 60 min (A=0.1% formic acid in water, B=0.1% formic acid in acetonitrile). The Q-Tof Premier (Waters, Inc.) was operated in the LC/MS E mode of acquisition, where alternating 2 s scans of low (4 V) or high (15−40 V) collision energies are used to generate either intact peptide ions (low energy) or peptide product ions (high energy). Each raw data file was processed using ProteinLynx Global Server (PLGS) V2.3 software (Waters, Inc.) to generate charge state reduced and deisotoped precursor mass lists as well as associated product ion mass lists for subsequent protein identification and quantification. Each processed file was searched against the Uniprot/Swissprot databases using the IDENTITY E database search algorithm within PLGS V2.4. Parameters were set to: peptide tolerance=15 p.p.m. ; fragment tolerance=30 p.p.m. ; minimum fragment ion matches per peptide=3; minimum fragment ion matches per protein=7; minimum peptide ion matches per protein=2; primary digest reagent=trypsin; missed cleavages=2; cysteine carbamidomethylation as fixed modification and methionine oxidation, asparagine and glutamine deamination as variable modifications. A false positive rate of 4% was allowed, and calculated by the appearance in search results of peptides from a randomized protein database [60] . Each sample was injected in triplicate and the data were pooled, and the expected fragments from iTRAQ labels were extracted. Peptides were included in study if there was a ladder score of >10, if they were identified as having an isobaric tag and if all four isobaric label fragments were present. Peptide relative quantification Values for the contribution of each isobaric tag were extracted from processed raw files and matched to the peptide identification. For each peptide, the ion intensity of the isobaric tag corresponding to the mock-dephosphorylated samples was divided by those of the in-vitro dephosphorylated samples. To normalize for errors in sample mixing, peptides identified as not containing serine, threonine or tyrosine (non-STY) were averaged for each of the FK506- or DMSO-treated samples. All peptides were then normalized to these values independently for the values arising from FK506- or DMSO-treated samples. To examine potential kinase sites, data from peptides containing the same S, T or Y residues were pooled, and an average was generated for each set of S, T or Y residues ( Supplementary Table 1 ). The Brg1 protein sequence was submitted to NetPhosK to identify potential kinase sites using a cutoff value 0.4. For each kinase, peptides were scored as targets if they contained a serine or threonine scoring above this threshold. Logistic regression was then used to determine the association between the presence of a kinase site and the ratio of isobaric labels from the FK506-treated samples. TiO 2 phosphopeptide enrichment Phosphopeptides were enriched using a NuTip TiO 2 micropipette tip (Glygen Corp.). The dried peptide digest was dissolved in 10 μl of binding solvent (75:19:6=acetonitrile/water/TFA) and on-third was used for enrichment. A 1–10 μl TiO 2 NuTip was washed two times with 10 μl aliquots of binding solvent. Phosphopeptides were bound by repetitive pipetting (20 times) of the 10 μl sample volume. The NuTip was then washed five times with binding solvent and then five times with 0.1% TFA. Phosphopeptides were then eluted in a separate tube with a 10-μl volume of 6% NH 4 OH after repetitive pipetting (10 times). A 5-μl aliquot of 5% TFA was then added and the phosphopeptides were further concentrated in a Speed Vac before injection on the LC-MS/MS system. LC-MS/MS on Orbitrap Velos Tryptic peptides were dissolved in 20 μl of 0.1% TFA and a 3.5-μl aliquot was directly injected onto a custom packed trap column (2 cm × 100 μm C18). Peptides were then eluted and sprayed from a custom packed emitter (75 μM × 25 cm C18) with a linear gradient from 100% solvent A (0.1% formic acid in 5% acetonitrile) to 35% solvent B (0.1% formic acid in acetonitrile) in 90 min at a flow rate of 300 nl min −1 on a Proxeon Easy nanoLC system directly coupled to a LTQ Orbitrap Velos mass spectrometer (Thermo Scientific). Data-dependent acquisitions were set up according to an experiment where full MS scans from 350 to 2,000 m / z were acquired in the Orbitrap at a resolution of 60,000 followed by 10 MS/MS scans acquired in the LTQ ion trap instrument. The raw data files were processed with Extract_ MSN (Thermo Scientific) into peak lists and then searched against the Mouse index of the SwissProt database using the Mascot Search engine ver. 2.3 (Matrixsciences, Ltd.). Parent mass tolerances were set to 10 p.p.m. and fragment mass tolerances were set to 0.5 Da. Data were searched for tryptic peptides, with a maximum of two missed cleavages and instrument mode set to electrospray ionization fourier transform ion cyclotron resonance (ESI-FTICR). The variable modifications of acetyl (protein N-term), STY phosphorylation, pyro glutamic for N-term glutamine, carbamidomethylation of cysteine and oxidation of methionine were used. Mascot search results were loaded into the Scaffold software (Proteome Software, Inc.) to compare sample results. How to cite this article: Nasipak, B. T. et al. Opposing calcium-dependent signalling pathways control skeletal muscle differentiation by regulating a chromatin remodelling enzyme. Nat. Commun. 6:7441 doi: 10.1038/ncomms8441 (2015).